Optofluidic sorting of material chirality by chiral light The lack of mirror symmetry, chirality, plays a fundamental role in physics, chemistry and life sciences. The passive separation of entities that only differ by their handedness without need of a chiral material environment remains a challenging task with attractive scientific and industrial benefits. To date, only a few experimental attempts have been reported and remained limited down to the micron scale, most of them relying on hydrodynamical forces associated with the chiral shape of the micro-objects to be sorted. Here we experimentally demonstrate that material chirality can be passively sorted in a fluidic environment by chiral light owing to spin-dependent optical forces without chiral morphology prerequisite. This brings a new twist to the state-of-the-art optofluidic toolbox and the development of a novel kind of passive integrated optofluidic sorters able to deal with molecular scale entities is envisioned. Harnessing material handedness is a topical challenge for many industries as it is a basic requirement towards the synthesis of drugs, additives or pesticides, to name a few. This implies the development of chiral sorting strategies that correspond to the ability to separate two entities that only differ by their handedness. Established chiral separation techniques at molecular scale are mostly based on the recognition of material chirality by another material that is designed to distinguish between the left- and right-handed versions of the entity to be sorted [1] , [2] . Instead, passive approaches free from such chiral recognition may also be considered, for instance by relying on transport phenomena, as discussed in the early 70s [3] . More recently, several options based on the coupling between translational and rotational mechanical degrees of freedom in fluid flows have been proposed [4] , [5] , [6] , [7] , [8] , [9] , [10] and realized down to the micron scale by using various kinds of chiral-shaped microparticles made of non-chiral media [11] , [12] , [13] . In addition, hydrodynamic propeller effects driven by rotating electric fields have also been considered theoretically [14] , [15] . This principle has been demonstrated only recently by using screw-shaped micrometre-sized particles made of non-chiral medium subjected to the action of a rotating magnetic field [16] . Merging microfluidic and field-induced options into an optofluidic chiral sorting scheme may offer new possibilities for a technology that arouses interest regarding present achievements and promising developments (see ref. 17 and corresponding Focus Issue). Despite a few theoretical proposals to achieve photoinduced chiral separation [18] , [19] , [20] , [21] , [22] , [23] , the realization of an optical chiral sorter is, however, missing so far. In this work, we experimentally demonstrate the passive optical separation, in a fluidic environment, of mirror-imaged chiral microparticles that differ only by opposite handedness by using chiral light fields. Importantly, the proposed optofluidic strategy does not require chiral-shaped microparticles and actually relies on the chirality of the medium, in contrast to previous experimental demonstrations of chiral sorting based on hydrodynamical effects [11] , [12] , [13] , [16] . Indeed, our method enables to sort material chirality by exploiting a universal feature of the light–matter interaction, namely the dependence of optical forces on the intrinsic handedness of matter and light. Principle To demonstrate our concept of chiral sorting by chiral light, we propose to use an optical field that consists of two counterpropagating circularly polarized collimated beams with opposite handedness Λ=±1 (so called helicity, namely the projection of the spin of a photon along its propagation direction) but equal power and waist. Then, let us consider a microsphere with spherically symmetric bulk material properties and assume that it passes perpendicularly through the latter two-beam configuration at constant velocity V 0 , say along the x axis. For a non-chiral material, the net optical force component exerted on the object along the propagation direction of the beams, say the z axis, is zero by virtue of cancelation of the two individual beam contributions. In the absence of additional external forces exerted on the particle, its trajectory is thus straight. In contrast, if the material is chiral, the force balance does not hold anymore and a non-zero net force, which originates either from circular birefringence or circular dichroism, is now exerted on the particle. This consequently leads to a curved trajectory in the ( x , z ) plane. Noteworthy the sign of the particle trajectory’s curvature is expected to be reversed by the change Λ→−Λ or χ →− χ , where χ =±1 refers to the material handedness, non-chiral media being associated with χ =0. Experimental framework In practice, we used spherical liquid crystal microscopic droplets immersed in the bulk of an isodense and isotropic host fluid (≈25 wt% aqueous glycerol solution, refractive index n ext =1.36, dynamic viscosity η =2 mPa s) in a glass capillary. The driving optical field is provided by two continuous-wave Gaussian laser beams with vacuum wavelength λ 0 =532 nm and waist w 0 ~50 μm. The experimental setup is sketched in Fig. 1 . Trajectories and velocities of individual droplets are experimentally retrieved by direct optical video imaging using a microscope objective (magnification × 20, numerical aperture NA=0.35). Choosing a droplet lying in the ( x , z ) plane and displacing the capillary at a constant velocity V 0 along the x axis, the chiral separation scenario described above can be verified. 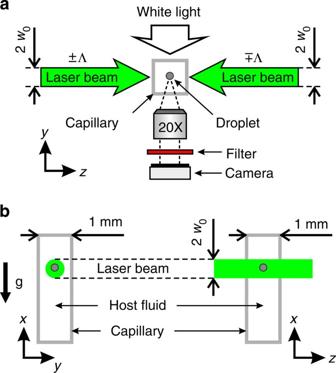Figure 1: Experimental setup. A droplet of radiusRand average refractive indexnis immersed in an aqueous glycerol solution of refractive indexnext<nin a glass capillary. (a) Top view. (b) Side view, wheregrefers to gravitational acceleration. The droplet is illuminated by two circularly polarized counterpropagating collimated Gaussian laser beams with opposite handedness (helicity Λ=±1), equal powerPand waistw0, at 532 nm wavelength. The droplet is imaged under white light illumination by means of a charge-couple device camera through a filter absorbing the laser radiation scattered from the sample. Figure 1: Experimental setup. A droplet of radius R and average refractive index n is immersed in an aqueous glycerol solution of refractive index n ext < n in a glass capillary. ( a ) Top view. ( b ) Side view, where g refers to gravitational acceleration. The droplet is illuminated by two circularly polarized counterpropagating collimated Gaussian laser beams with opposite handedness (helicity Λ=±1), equal power P and waist w 0 , at 532 nm wavelength. The droplet is imaged under white light illumination by means of a charge-couple device camera through a filter absorbing the laser radiation scattered from the sample. Full size image In present work, we used chiral (cholesteric) or non-chiral (nematic) liquid crystal spherical droplets having an overall radial structure of the director field n , which is a unit vector directed along the average local orientation of the liquid crystal molecules, as illustrated in Fig. 2a,b (see Methods for details regarding the nature and preparation of the droplets). The nematic droplets have a radial ordering of the director, whereas the cholesteric droplets are characterized by a helical order with pitch p (that is, the distance over which n rotates by 2 π ) and have a radial distribution of the helical axes. This radial symmetry formally saves us from the alignment of the droplet with respect to the beam axis. In practice, such symmetry is confirmed by a fourfold intensity pattern when imaging the droplets between crossed linear polarizers as shown in Fig. 2c,f . 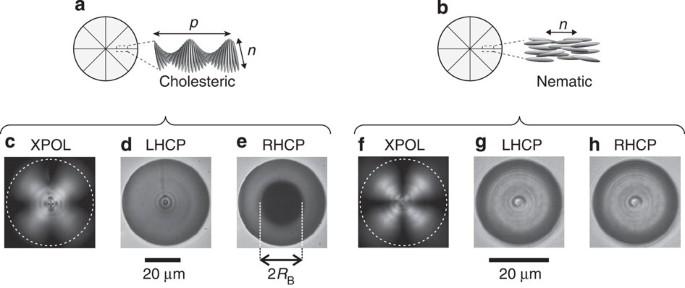Figure 2: Chiral and non-chiral liquid crystal radial droplets used in the present study. (a,b) Sketches of the director field for the chiral (cholesteric) and non-chiral (nematic) liquid crystal radial droplets that have been used in the present study, where the double arrow for the director refers to the equivalence ofnand −n. (c,f) Images of the droplets viewed between crossed linear polarizers (XPOL), where the fourfold patterns characterize the overall radial ordering of the droplets and the dashed circles refer to the contour of the droplets. (d,g) Images of the droplets under left-handed circularly polarized (LHCP) illumination. (e,h) Images of the droplets under right-handed circularly polarized (RHCP) illumination. Illumination wavelength: 532 nm. Scale bar: 20 μm (c–h). Figure 2: Chiral and non-chiral liquid crystal radial droplets used in the present study. ( a , b ) Sketches of the director field for the chiral (cholesteric) and non-chiral (nematic) liquid crystal radial droplets that have been used in the present study, where the double arrow for the director refers to the equivalence of n and − n . ( c , f ) Images of the droplets viewed between crossed linear polarizers (XPOL), where the fourfold patterns characterize the overall radial ordering of the droplets and the dashed circles refer to the contour of the droplets. ( d , g ) Images of the droplets under left-handed circularly polarized (LHCP) illumination. ( e , h ) Images of the droplets under right-handed circularly polarized (RHCP) illumination. Illumination wavelength: 532 nm. Scale bar: 20 μm ( c – h ). Full size image Sensitivity of the chiral droplets to the helicity of the driving light field is illustrated in Fig. 2d,e that show distinct images for the same droplet observed under left- and right-handed circularly polarized illumination at wavelength λ 0 , whereas the non-chiral droplets exhibit identical images as shown in Fig. 2g,h . More precisely, the black circular area of radius R B for the chiral droplet shown in Fig. 2e corresponds to the circular Bragg reflection phenomenon, which is a generic optical property of cholesteric liquid crystals [24] . It refers to the fact that the propagation of light in one of the two circular polarization states along the cholesteric helical axis is forbidden over a well-defined wavelength range Δ λ = p(n ∥ −n ⊥ ) centred on the Bragg wavelength λ B = np where n=(n ∥ −n ⊥ )/2 is the average refractive index of the cholesteric with n ∥ , ⊥ the refractive indices parallel and perpendicular to n . By deliberately choosing Bragg cholesteric droplets, enhanced optomechanical separation of droplets having opposite chirality is achieved at relatively low optical power due to helicity-dependent optical radiation pressure exerted on the droplets [25] . Experimental proof-of-principle The experimental demonstration of optical chiral sorting is illustrated in Fig. 3 , where panels 2 a – c depict the light–matter interaction geometry, whereas panels 2d-f compile snapshots of the droplet dynamics for Λ χ =−1, χ =0 and Λ χ =+1, respectively, where χ =0 refers to the control experiment with a non-chiral radially ordered droplet. Due to the bounded nature of the light beams, a chiral droplet experiences a finite displacement along z , namely Δ z = z +∞ − z −∞ , as depicted in Fig. 3d,f . Here z ±∞ refers to the z coordinate of the droplet centre of mass at time t = t ±∞ , with t=0 when the droplet crosses the beam axis at x =0. In contrast, a non-chiral radial nematic droplet is not deviated while passing across the beams, as shown in Fig. 3e . Clearly, the fact that Δ z is proportional to Λ χ demonstrates the possibility to sort objects with different chirality by chiral light. 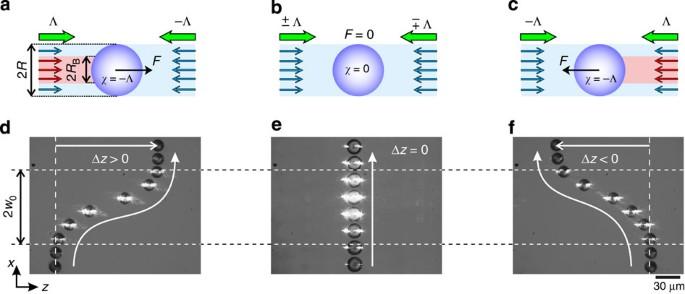Figure 3: Optical sorting of droplets with different chirality. (a,b,c) Different light–matter interaction geometries, where two kinds of contributions to the net optical forceFare identified for Bragg chiral droplets: red arrows refer to the ‘Bragg optical rays’ that are considered to be totally reflected due to circular Bragg reflection over a circular cross-section of radiusRB(visualized inFig. 2e), whereas blue arrows refer to the ‘Fresnel optical rays’ that are considered to be refracted/reflected on the droplet as is the case for an isotropic non-chiral dielectric sphere. (d–f) Demonstration of passive chiral optical sorting concept with chiral (d,f) and non-chiral (e) droplets that pass perpendicularly through the beams at a constant velocityV0along thexaxis. The pictures are obtained by superimposing snapshots taken at a discrete set of time. Only chiral droplets experience a non-zero deviation Δzalong thezaxis that is proportional to Λχ, whereχ=0 refers to non-chiral medium andχ=±1 to right/left-handed chiral media. Parameters: beam power isP=170 mW, beam waistw0≈50 μm, driving velocity isV0=12 μm s−1. Scale bar: 30 μm (d–f). Figure 3: Optical sorting of droplets with different chirality. ( a , b , c ) Different light–matter interaction geometries, where two kinds of contributions to the net optical force F are identified for Bragg chiral droplets: red arrows refer to the ‘Bragg optical rays’ that are considered to be totally reflected due to circular Bragg reflection over a circular cross-section of radius R B (visualized in Fig. 2e ), whereas blue arrows refer to the ‘Fresnel optical rays’ that are considered to be refracted/reflected on the droplet as is the case for an isotropic non-chiral dielectric sphere. ( d – f ) Demonstration of passive chiral optical sorting concept with chiral ( d , f ) and non-chiral ( e ) droplets that pass perpendicularly through the beams at a constant velocity V 0 along the x axis. The pictures are obtained by superimposing snapshots taken at a discrete set of time. Only chiral droplets experience a non-zero deviation Δ z along the z axis that is proportional to Λ χ , where χ =0 refers to non-chiral medium and χ =±1 to right/left-handed chiral media. Parameters: beam power is P =170 mW, beam waist w 0 ≈50 μm, driving velocity is V 0 =12 μm s −1 . Scale bar: 30 μm ( d – f ). Full size image Importantly, optofluidic chiral sorting is not restricted to resonant chiral interaction as is the case for Bragg chiral droplets. Indeed it works for non-Bragg radial cholesteric droplets as well. This is demonstrated in Fig. 4 that presents the case of left- and right-handed radial cholesteric droplets with p ≈2 μm (see Methods for details). Such droplets indeed do not exhibit circular Bragg reflection phenomenon as demonstrated by comparing the images of the droplet under LHCP and RHCP illumination, see Fig. 4a–d , where the material chirality reveals itself as spiralling texture in the images. Even if the optomechanical effect is visible ( Fig. 4e,f ), the light-induced deviation is typically 20 times smaller than the one obtained in the Bragg case when considering identical optical power, flow velocity and droplet radius. This basically results from the fact that the helicity-dependent scattering of light by non-chiral microparticles is not a resonant process, in contrast to circular Bragg reflection. In this regard, we note a recent theoretical study on optical forces exerted on isotropic chiral spherical scatterers [26] . 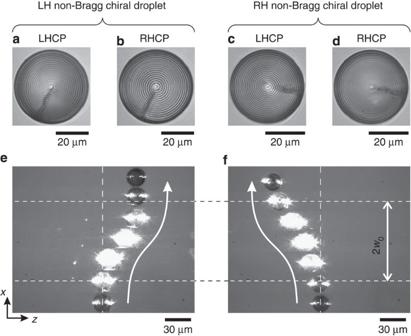Figure 4: Sorting radial cholesteric droplets. The sorting is done by chiral light without relying on circular Bragg reflection phehomenon. Upper panels: image under LHCP (a,c) and RHCP (b,d) illumination at 532 nm wavelength of left- and right-handed radial cholesteric droplets having a pitchp≈2 μm. Bottom panels: optical sorting experiments for left-handed (e) and right-handed (f) droplets. The sign of the optically induced deviation along thezaxis depends on the material chirality at fixed interaction geometry, thereby extending the proposed optofluidic chiral sorting scheme to non-Bragg chiral micro-objects. Parameters: beam power isP=540 mW, beam waist isw0≈50 μm, driving velocity isV0=12 μm s−1. Scale bar: 20 μm (a–d) and 30 μm (e,f). Figure 4: Sorting radial cholesteric droplets. The sorting is done by chiral light without relying on circular Bragg reflection phehomenon. Upper panels: image under LHCP ( a , c ) and RHCP ( b , d ) illumination at 532 nm wavelength of left- and right-handed radial cholesteric droplets having a pitch p ≈2 μm. Bottom panels: optical sorting experiments for left-handed ( e ) and right-handed ( f ) droplets. The sign of the optically induced deviation along the z axis depends on the material chirality at fixed interaction geometry, thereby extending the proposed optofluidic chiral sorting scheme to non-Bragg chiral micro-objects. Parameters: beam power is P =540 mW, beam waist is w 0 ≈50 μm, driving velocity is V 0 =12 μm s −1 . Scale bar: 20 μm ( a – d ) and 30 μm ( e , f ). Full size image Put together, all these observations unambiguously demonstrate that a reliable optical sorting of material chirality can be achieved. Indeed, as shown in Fig. 1 , one easily gets Δ z ≫ R within a few seconds and with 100% efficiency. Typically we thus have Δ z≈R in one second using P =10 mW and V 0 =10 μm s −1 . Moreover, the obtained dependencies of Δ z on (i) optical chirality at fixed material chirality ( Fig. 3 ) and (ii) material chirality at fixed optical chirality ( Fig. 4 ) fully demonstrate an optofluidic chiral sorting that is basically associated with light-induced separation scaling as Δ z ∝ Λ χ . Quantitative analysis We have also studied the optical sorting process versus the driving velocity V 0 and the beam power P in the Bragg case. We found that larger the P is at fixed V 0 , the larger is Δ z , whereas larger the V 0 is at fixed P , the smaller is Δ z . Quantitatively, one obtains Δ z = a ( P / V 0 ), a being a constant, as demonstrated in Fig. 5a that gathers the results of 48 independent realizations for a radial cholesteric droplet with radius R =15 μm and where the solid line refers to the best linear fit. More quantitatively, the best fit slope value a =31.8 nm N −1 can be compared with the predictions for the net optical force exerted on the droplet based on a ray-optics model (see Supplementary Figure 1 for illustration), by calculating the net change of linear momentum of the light field as it interacts with the droplet, which is done by attributing the Minkowski linear momentum ℏ k ( ℏ is the reduced Planck constant, k the wavevector magnitude) per photon pointing along each geometrical ray. 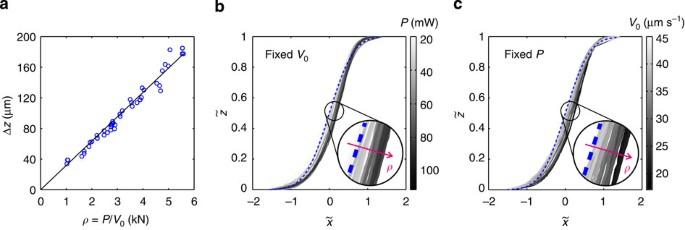Figure 5: Light-induced spatial separation and universality of the sorting trajectories. (a) Experimental droplet deviation along thezaxis, Δz, as a function of the parameterρ=P/V0for 48 independent realizations. Solid line is the best linear fit passing through the origin, as predicted by our model, seeSupplementary Information. (b,c) Reduced trajectories in the coordinate systemwhenPis varied at fixed velocityV0=17 μm s−1(b) and whenV0is varied at fixed powerP=95 mW (c). Enlargement windows point out the trend as the parameterρincreases: the larger isρ, the more the droplet trajectories depart from the universal trajectory given by the normal cumulative distribution function, here represented by dashed curves. Parameters: beam waist isw0≈50 μm and droplet radius isR=15 μm. Figure 5: Light-induced spatial separation and universality of the sorting trajectories. ( a ) Experimental droplet deviation along the z axis, Δ z , as a function of the parameter ρ = P / V 0 for 48 independent realizations. Solid line is the best linear fit passing through the origin, as predicted by our model, see Supplementary Information . ( b , c ) Reduced trajectories in the coordinate system when P is varied at fixed velocity V 0 =17 μm s −1 ( b ) and when V 0 is varied at fixed power P =95 mW ( c ). Enlargement windows point out the trend as the parameter ρ increases: the larger is ρ , the more the droplet trajectories depart from the universal trajectory given by the normal cumulative distribution function , here represented by dashed curves. Parameters: beam waist is w 0 ≈50 μm and droplet radius is R =15 μm. Full size image Although we refer to Supplementary Note 1 for details regarding the derivation of the model, the main result is worth to be mentioned. Namely, assuming that the beam propagating towards z >0 is associated with Λ χ =−1, the z component of the net optical force exerted on the droplet can be approximated by where the x coordinate is the distance from the droplet centre of mass to the propagation axis of the two beams, c is the speed of light in vacuum and θ B,ext =arcsin( R B / R ) is the half-apex angle of the cone that defines the circular cross-section of radius R B for which the droplet is assumed to behave as a perfect curved mirror (see Supplementary Figure 2 ). We notice that such an angle is related to the angle θ B =arcsin[( n ext / n )sin θ B,ext ], which is an intrinsic characteristic of the cholesteric medium that depend neither on the droplet radius nor on the refractive index of the host fluid. In the limit of small Reynolds number, as is the case in our experiments, the expression for the light-induced droplet velocity is then obtained from the balance between the viscous force exerted by the surrounding fluid on the moving droplet and the driving optical force. The z component of the droplet velocity thus expresses as There is also a non-zero component of the optical force along the x axis, F x ( x ), whose cumbersome expression can be found in Supplementary Information . The ensuing light-induced x component for the droplet velocity is written v x ( x )= F x ( x )/(6 πηR ). The total droplet velocity along x therefore expresses as V x ( x )= V 0 + v x ( x ). Once the expression of the force exerted on the droplet is determined, the droplet trajectory can be retrieved, which is the key feature of the optical sorting. This is done by noting that V x ( x )=d x /d t and v z ( x )=d z /d t , from which one gets d z = v z ( x )/( v x ( x )+ V 0 )d x . Integration of d z along the x axis thus gives access to the droplet trajectory z ( x ) and total deviation Δ z . In particular, under the approximation v x << V 0 one gets where we recognize the factor introduced above as the slope of the linear fit shown in Fig. 5a . Taking θ B,ext as the only adjustable parameter, we obtain θ B,ext =25.1±1.1°, hence θ B =21.3±0.9° ( n ext =1.36 and n =1.60), which fairly agrees with a previous measurement [25] . Remarkably, when Equation (1) is valid and under the approximation v x ≪ V 0 , the expression of the droplet trajectory simplifies to where Φ is the normal cumulative distribution function, By introducing the reduced coordinates and , the droplet trajectory adopts the universal expression . This is demonstrated in Fig. 5 where the universal trajectory is displayed as a dashed line. In this figure, the experimental reduced trajectories as a function of P at fixed V 0 are shown in Fig. 5b , whereas those as a function of V 0 at fixed P are shown on Fig. 5c . Still, slight deviations from the universal behaviour, with a clear trend, are identified within the presented range of parameters for V 0 and P . This is qualitatively illustrated by the insets of Fig. 5b,c . Namely, the larger is the parameter ρ = P / V 0 , the larger is the deviation from the universal behaviour. A more quantitative assessment of it is presented in Fig. 6a that displays the reduced distance from the beam axis at versus the reduced parameter ξ = ρ / ρ c . Here ρ c is the critical value of ρ above which a droplet is eventually trapped by light and consequently guided along the z axis towards the ± z direction depending on the sign of Λ χ , whereas the transverse location of the droplet centre is constant. Using actual experimental parameters and R =15 μm, we numerically find ρ c =9.66 kN, which typically corresponds to P =100 mW and V 0 =10 μm s −1 . In fact, these predictions regarding the trapping regime fit well our observations as the experimental data presented in Fig. 5a indeed fall in the range 0.1< ξ <0.6, hence dealing with the chiral sorting regime without trapping. The quantitative agreement with the model (accounting for both F x and F z ) is emphasized by the solid curve in Fig. 6a . Moreover, for the sake of a thorough presentation of the two regimes, a few simulated trajectories for various values of the reduced parameter ξ = ρ / ρ c are shown in Fig. 5b both in the sorting ( ξ <1) and trapping ( ξ >1) cases. 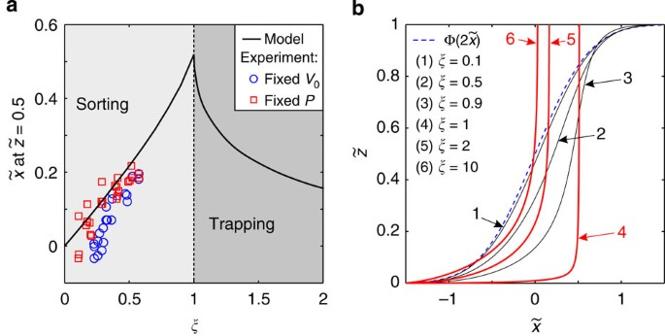Figure 6: Optical sorting versus optical trapping. (a) Reduced distanceof the droplet from the beam axis atfor all the data shown inFig. 5b,c. Solid curve refers to simulations. (b) Simulated reduced trajectories as a function of the reduced parameterξ=ρ/ρc(see text for details). The droplet follows the typical behaviour shown inFig. 5b,cwhenξ<1, whereas the droplet is eventually trapped at a constantin the path of the beams and consequently guided along thezaxis whenξ>1. Figure 6: Optical sorting versus optical trapping. ( a ) Reduced distance of the droplet from the beam axis at for all the data shown in Fig. 5b,c . Solid curve refers to simulations. ( b ) Simulated reduced trajectories as a function of the reduced parameter ξ =ρ/ρ c (see text for details). The droplet follows the typical behaviour shown in Fig. 5b,c when ξ <1, whereas the droplet is eventually trapped at a constant in the path of the beams and consequently guided along the z axis when ξ >1. Full size image The reliability of our experimental approach and its quantitative description are further emphasized by looking at the droplet dynamics in the sorting regime. Its statistical analysis is presented in Fig. 7a,b where the longitudinal and the transverse light-induced droplet velocity components v z and v x , divided by P for the sake of universalization, are presented for the data shown in Fig. 5a . 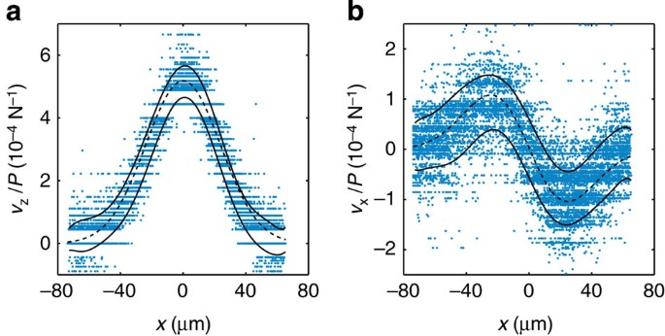Figure 7: Droplet dynamics in the sorting regime. Experimental longitudinal (a) and transverse (b) light-induced droplet velocity components (divided byP) during the optical chiral sorting dynamics for the 48 dataset used inFig. 5a. Markers are experimental data, solid curves outline the experimental standard deviation range and dashed curves refer to simulations. Figure 7: Droplet dynamics in the sorting regime. Experimental longitudinal ( a ) and transverse ( b ) light-induced droplet velocity components (divided by P ) during the optical chiral sorting dynamics for the 48 dataset used in Fig. 5a . Markers are experimental data, solid curves outline the experimental standard deviation range and dashed curves refer to simulations. Full size image The obtained quantitative agreement between our observations and our model (which neglects absorption) without need for adjustable parameters eliminates the possibility that thermal effects are at the origin of the reported effects. Also, this demonstrates that the reported optical sorting scheme is immune to unavoidable (according to the hairy ball theorem) presence of a radial defect in radial cholesteric droplets [27] , [28] that formally breaks the spherical symmetry of the radial cholesteric droplets, as shown in Fig. 2d for Bragg droplets and in Fig. 4a–d for non-Bragg ones. This emphasizes the generality of the reported results on optofluidic sorting of chiral microparticles by chiral light. A natural extension of the present work would consist in the downsizing from the micron scale down to the molecular scale. Indeed, despite an obvious practical interest there are only a few theoretical works dealing with electromagnetic field-induced mechanical separation of nanometre-sized chiral entities [14] , [15] , [18] , [19] , [20] , [21] , [22] , [23] , whereas no experimental realization has been reported so far. However, straightforward downsizing of an approach based on the circular Bragg reflection phenomenon has obvious inherent limitations. Indeed the formation of Bragg droplets requires a droplet diameter sufficiently larger than the pitch, which scales as the wavelength and thus prevents from considering sub-micrometric droplets. Outside the resonance, optomechanical effects are less efficient, as experimentally shown here in Fig. 4 , and are thus expected to be more sensitive to thermal noise. To overcome this limitation, one might consider an alternative strategy that combines robustness and efficiency of the optomechanically resonant Bragg approach with material chiral recognition applied in standard separation techniques, as sketched in Fig. 8 . In that case, chiral microparticles act as ‘conveyers’ whose appropriate surface functionalization allows sorting chiral or non-chiral entities at molecular scale. Of course, solid Bragg chiral microparticles would be desirable for this purpose and protocols actually exist to fabricate them [29] . In addition, large-scale accurate fabrication of photopolymerized Bragg chiral conveyers can be considered exploiting microfluidic preparation protocols [30] . 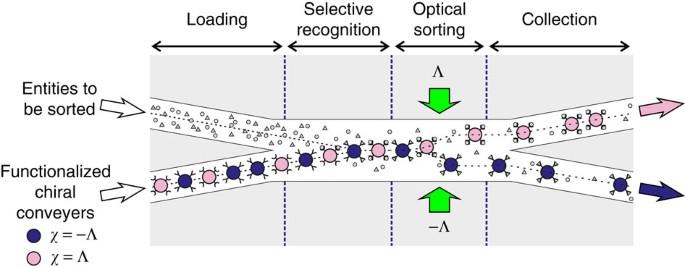Figure 8: Illustration of an integrated optofluidic sorter. The microfluidic version of the proposed optical chiral sorting scheme is expected to process any random sequence of left-handed and right-handed chiral microparticles, for instance using a Y-shaped bifurcating microfluidic output channel. Moreover, chiral microparticles may also be used as ‘chiral conveyers’ for molecular scale entities. When mixed with small scale entities to be sorted, chiral conveyers with appropriate functionalization may selectively bind their target in the fluidic environment, then be sorted by light and eventually collected in two different output microchannels. Figure 8: Illustration of an integrated optofluidic sorter. The microfluidic version of the proposed optical chiral sorting scheme is expected to process any random sequence of left-handed and right-handed chiral microparticles, for instance using a Y-shaped bifurcating microfluidic output channel. Moreover, chiral microparticles may also be used as ‘chiral conveyers’ for molecular scale entities. When mixed with small scale entities to be sorted, chiral conveyers with appropriate functionalization may selectively bind their target in the fluidic environment, then be sorted by light and eventually collected in two different output microchannels. Full size image To conclude, these results present the first experimental demonstration of passive optical sorting of material chirality. As chiral sorting strategies have a huge application potential, we anticipate that this study will promote further developments of the existing optofluidic toolbox [31] , [32] . It may also contribute to the emergence of other kinds of field-induced chiral sorting strategies more generally based on the use of angular momentum of light, be it of spin or orbital nature. Preparation of liquid crystal droplets Radial nematic droplets are obtained by dispersing the nematic E7 (from Merck) in water with a small fraction (0.2 g l −1 ) of surfactant CTAB (cetyltrimethylammonium bromide, from Sigma-Aldrich) that promotes a perpendicular alignment of n at the nematic/water interface. On the other hand, radial cholesteric droplets are obtained by dispersing the material in an aqueous glycerol solution that promotes a parallel alignment for the director at the cholesteric/fluid interface, hence a radial distribution of the cholesteric helix axes. The solution contains ≈25 wt% of glycerol in order to get an isodense emulsion. Different cholesteric mixtures have been used: (i) the nematic E7 doped with ≈5 wt% of either left-handed S811 or right-handed dopant R811 (both from Merck), which give p ≈2 μm and (ii) the cholesteric mixture MDA-02-3211 (from Merck) with pitch p =347nm at room temperature. How to cite this article: Tkachenko, G. & Brasselet, E. Optofluidic sorting of material chirality by chiral light. Nat. Commun. 5:3577 doi: 10.1038/ncomms4577 (2014).